Flexible and low-voltage integrated circuits constructed from high-performance nanocrystal transistors Colloidal semiconductor nanocrystals are emerging as a new class of solution-processable materials for low-cost, flexible, thin-film electronics. Although these colloidal inks have been shown to form single, thin-film field-effect transistors with impressive characteristics, the use of multiple high-performance nanocrystal field-effect transistors in large-area integrated circuits has not been shown. This is needed to understand and demonstrate the applicability of these discrete nanocrystal field-effect transistors for advanced electronic technologies. Here we report solution-deposited nanocrystal integrated circuits, showing nanocrystal integrated circuit inverters, amplifiers and ring oscillators, constructed from high-performance, low-voltage, low-hysteresis CdSe nanocrystal field-effect transistors with electron mobilities of up to 22 cm 2 V −1 s −1 , current modulation >10 6 and subthreshold swing of 0.28 V dec −1 . We fabricated the nanocrystal field-effect transistors and nanocrystal integrated circuits from colloidal inks on flexible plastic substrates and scaled the devices to operate at low voltages. We demonstrate that colloidal nanocrystal field-effect transistors can be used as building blocks to construct complex integrated circuits, promising a viable material for low-cost, flexible, large-area electronics. Colloidal semiconductor nanocrystals (NCs) are prized for their size- and shape-tunable electronic properties [1] , [2] , [3] , [4] . Wet-chemical methods have enabled the preparation of highly uniform, monodisperse crystalline NCs for a wide variety of chemical compositions by commonly employing long-chain organic ligands to control NC synthesis and to stabilize NC dispersions [5] . These NC solutions capped with long ligands can be easily processed by a variety of solution-based material deposition methods (spincasting, dipcoating, inkjet printing, dropcasting, spraycoating) to form uniform thin films [6] , [7] , [8] , [9] , [10] , [11] . Although high-quality NC synthesis and dispersibility relies on long ligands, these ligands are insulating and prevent strong coupling and charge transport between NCs once assembled in the solid state. Until recently, this has posed a significant challenge to using these colloidal inks as technologically viable electronic materials for devices [12] and integrated circuitry [13] . Advances in ligand chemistry have shown that the original, long ligands used in synthesis can be replaced by shorter inorganic ligands [14] , [15] , [16] , [17] either in solution, and still maintain solution dispersibility and thin-film processability, or in thin-film solids. These novel ligands preserve the discrete, size-dependent features of quantum confinement and enhance electronic coupling between the NCs in thin films. Our group, along with the Talapin group, have shown that dispersions of NCs exchanged with compact ligands can be spincast to form dense, crack-free, thin films that demonstrate excellent performance in single field-effect transistors (FETs), with high electron mobilities exceeding 15 cm 2 V −1 s −1 (refs 16 , 18 , 19 , 20 ). The solution processability and high performance of NC-FETs make colloidal NC semiconductors extremely attractive as colloidal inks for low-cost, large-scale coating and printing of thin-film electronics. Although there has been significant progress in developing single high-mobility NC-FETs that further operate with low hysteresis [18] , [20] at low voltage 19 , these high-performance NC-FETs have not been integrated into NC circuits in the literature. All circuit demonstrations have been limited to two single separate FETs connected externally to form an inverter [19] , [21] . To realize NC integrated circuits (NCICs) for large-area, thin-film electronics, it is necessary to go beyond discrete FET fabrication, to integrate multiple FETs into circuits and to evaluate device operation, such as the switching speed and signal amplification of the NC-FET. This requires that NC thin films be processed and deposited over a large area to form uniform devices that operate in concert as circuits. Here we report the first NCIC inverters, amplifiers and ring oscillators fabricated from high-mobility CdSe NC-FETs. We previously introduced high-mobility CdSe NC-FETs that operated at high voltages on rigid substrates, achieved through both strong coupling, by introducing the compact ligand ammonium thiocyanate, and through doping, by thermal diffusion of indium at mild temperatures [20] . Thiocyanate is an environmentally benign and non-corrosive ligand, allowing solution deposition of NC devices on a variety of substrates, including flexible plastic substrates, which we have previously demonstrated [21] . This greatly expands the applicability of these materials compared with other recently developed novel ligands. For example, although excellent mobilities have been observed with molecular metal chalcogenide complexes [18] , [19] , these NCs are dissolved in hydrazine, an extremely caustic solvent that is not compatible with flexible plastics. In addition, as a wide range of flexible electronic applications are typically powered by small thin-film batteries or radio frequency fields [22] , [23] , it is necessary to show the scalability of these colloidal inks to minimize energy consumption. We recently demonstrated low-voltage operation of flexible colloidal nanowire FETs using thin Al 2 O 3 as our robust, high capacitance and low-leakage gate dielectric material compatible with plastics [24] . In this work, we demonstrate high-performance NC-FETs that operate at low voltages on flexible plastics and serve as the building blocks of complex integrated circuits, demonstrating this class of materials as a viable, flexible electronic technology. Flexible and low-voltage NC-FETs To fabricate flexible devices, we used either a 25- or 50-μm thick polyimide substrate and covered the substrate with 30 nm of atomic layer deposited (ALD) Al 2 O 3 at 250 °C. Encapsulation with Al 2 O 3 preshrinks the polyimide substrate before subsequent thermal processing, which would otherwise cause severe delamination and cracking of the deposited NC thin films and metal electrodes. A 20-nm thick Al back gate was deposited by thermal evaporation through a shadow mask. The device was exposed to an oxygen plasma to increase the thickness of the native Al 2 O 3 on the Al gate and to create additional hydroxyl groups necessary for subsequent growth of a 30-nm ALD Al 2 O 3 gate dielectric layer. The measured capacitance of the dielectric layer was 0.253±0.019 μF cm −2 , allowing for low-voltage operation. We also characterized the FET gate leakage at pA levels to verify that current modulation arose from the CdSe NC thin-film channel and to show that the thin layer of ALD Al 2 O 3 formed a robust gate oxide that is suitable for use in flexible electronics ( Supplementary Fig. S1 ). To prepare the NC dispersion for spincoating, monodisperse CdSe NCs with as-synthesized long insulating ligands were treated in solution with ammonium thiocyanate in a nitrogen glovebox [16] , [20] , replacing the long ligands with the compact thiocyanate ligands, while maintaining solution dispersibility. The thiocyanate-exchanged NCs were redispersed in dimethylformamide and spincast atop the flexible substrates to form uniform, crack-free, randomly close-packed NC thin-film semiconducting channels. Unlike organic semiconductors, where the morphology and mobility of the material is reported to be highly dependent on the surface roughness [25] , we found that the NC thin films are largely insensitive to a root-mean-squared value as large as a couple of nanometres. Inside a nitrogen glovebox with an integrated evaporator, In/Au (50 nm/40 nm) electrodes were thermally deposited through a shadow mask atop the NC thin film to complete back-gate/top-contact FETs ( Fig. 1a ). We have also fabricated back-gate/bottom-contact devices, but these devices typically suffer from larger contact resistance and therefore display poorer device performance ( Supplementary Fig. S2A–C ). For the back-gate/top-contact FETs, typical output (drain current versus drain-source voltage ( I D − V DS ); Fig. 1c ) characteristics show n -type device behaviour that is modulated by a small positive voltage as low as 2 V. The extracted electron FET mobilities from the transfer curves (drain current versus gate voltage ( I D − V G ); Fig. 1d and Supplementary Methods ) in the linear regime ( V DS =0.1 V) are 21.9±4.3 cm 2 V −1 s −1 and in the saturation regime ( V DS =2 V) are 18.4±3.6 cm 2 V −1 s −1 . We translated our previous work on high-performance CdSe NC-FETs on rigid wafers operating at high voltages [20] to plastic substrates operating at low voltages. These FETs show high I ON / I OFF over 10 6 , low subthreshold swing ( S =0.28±0.09 V dec −1 ), low threshold voltage ( V T =0.38±0.15 V) and low hysteresis (Δ V T =0.25±0.07 V) at V DS =2 V. We attribute the low hysteresis to passivation of the NC surface by indium and the selection of Al 2 O 3 as the gate dielectric material, which we have shown to reduce the density of trap states at the NC surface and at the semiconductor-gate dielectric interface that give rise to hysteresis in NC-FETs. [20] As such, the small variation in device parameters and large-area uniformity of these NC-FETs enables their integration in flexible NCICs. 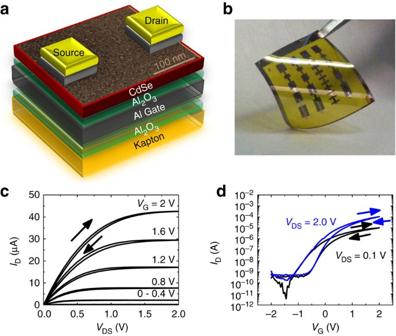Figure 1: Flexible CdSe NC-FETs. (a) Schematic and (b) photograph of a flexible CdSe NC-FET atop a Kapton substrate. (c) OutputID–VDSand (d) transferID−VGcharacteristics of a flexible, CdSe NC-FET. Figure 1: Flexible CdSe NC-FETs. ( a ) Schematic and ( b ) photograph of a flexible CdSe NC-FET atop a Kapton substrate. ( c ) Output I D – V DS and ( d ) transfer I D − V G characteristics of a flexible, CdSe NC-FET. Full size image Flexible NCICs To demonstrate the applicability of these high-performance, flexible CdSe NC-FETs as building blocks in integrated circuits, we constructed n -type unipolar inverters, amplifiers and ring oscillators, and studied their basic parameters for analogue and digital circuit applications. Similar to our fabrication of flexible NC-FETs, circuits were fabricated on either 25- or 50-μm thick preshrunk, Al 2 O 3 encapsulated polyimide substrates with thermally deposited 20-nm Al gate patterns, but here we developed a simple, additive process for Au-filled vertical interconnect access (VIA) holes to integrate device layers. This VIA process is unlike those previously developed through Al 2 O 3 that required corrosive and subtractive etching [26] , [27] . A VIA shadow mask was microscopically aligned to the Al gate lines and 60 nm of Au was thermally deposited to pattern the VIAs. The sample (with both gate and VIAs) was then exposed to an oxygen plasma to selectively increase the thickness of the native Al 2 O 3 atop the Al lines, which only grows an unstable oxide atop Au [28] , [29] . ALD Al 2 O 3 then selectively deposits a high-quality oxide atop the Al, but not atop the Au, which still retains conductivity after ALD, as experimentally verified. Thiocyanate-exchanged CdSe NCs were then spincast uniformly atop the samples, followed by thermal evaporation of In/Au electrodes through a shadow mask to form different integrated circuit topologies. 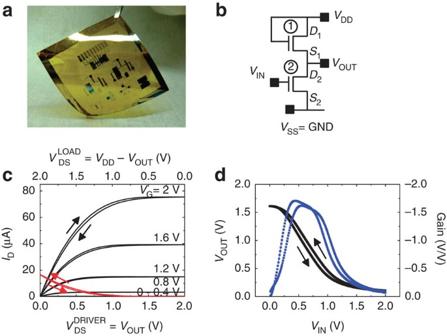Figure 2: Flexible NCIC inverter constructed from NC-FETs. (a) Photograph and (b) circuit schematic of saturated load inverters. (1) Load NC-FET and (2) driver NC-FET. (c) Graphical analysis of constituent driver (black) and load (red) NC-FET output characteristics, sweeping in forward and reverse, comprising the NCIC inverter, and (d) the corresponding voltage transfer characteristics (black, left axis) and gain characteristics (blue, right axis) of the NCIC inverter sweeping forward and reverse at a supply voltage of 2 V (VDD). GND, ground. NC integrated inverters Figure 2a shows an optical micrograph of solution-deposited CdSe NCIC inverters fabricated on flexible plastics substrates. The fabricated integrated inverters are based on a saturated load design as depicted in the circuit layout ( Fig. 2b ), where one n -type FET acts as an active load and the other n -type FET as a driver. As the threshold voltage is positive and the drain and gate voltages are identical, the load FET always operates in saturation. Our CdSe NCIC inverters were designed to have a driver with channel length ( L ) and width ( W ) ratio of 40 ( L =40 μm, W =1,600 μm), and to have a load with W / L of 10 ( L =40 μm, W =400 μm). We measured the output characteristics of the constituent driver and load FETs of the inverter element separately to insure that they operated as designed ( Fig. 2c ). The on-current for the driver is approximately four times larger than that for the load, as expected from the ratio of channel W/L . Graphical analysis ( Fig. 2c and Supplementary Fig. S3A ) provides a construction of the voltage transfer characteristic (VTC) of our integrated inverter from the constituent NC-FET building blocks. A representative VTC measured from a fabricated, flexible integrated inverter emulates the constructed VTC ( Fig. 2d ) and Supplementary Fig. S3B ). The inverter gets its name from inverting a ‘low’ input signal to a ‘high’ output signal, and a ‘high’ input signal to a ‘low’ output signal. For multiple flexible inverters, VTCs show a 1.5±0.1 V output swing, which makes use of 75% of the available supply voltage ( V DD =2 V). The output swing is consistent with that expected for the saturated load design, where the voltage output high is limited by the FET threshold voltage to the difference between supply and threshold voltages V DD − V T . Our inverters show voltage amplification with gains averaging −1.58±0.26 V/V, reaching as high as the theoretical gain of −2 V/V. The maximum gain of −2 V/V is consistent with that expected for a metal-oxide semiconductor common-source amplifier with a saturated load, defined by the channel dimensions of the constituent FETs (ref. 30 ), and may be tailored by choice of the load and driver geometries, depending on the design specification. The low hysteresis in the inverter VTC is ascribed to hysteresis in the NC-FET characteristics. The inverters’ VTCs show wide, linear regions of gain, allowing for input signal amplification and inversion of logic output high and low at the extremes of the VTCs, enabling signal switching. On the other hand, owing to the large input resistance (0.5 TΩ) and relatively low output resistance (few tens of kΩ; Supplementary Fig. S1 and Discussion), these amplifiers could also serve as a buffer stage in circuitry. The inverter is the most basic element in circuits used to construct amplifiers for analogue circuits and logic gates for digital circuits. The NCIC inverters’ VTCs follow circuit design expectations with wide output swing and proper gain, and show adequate noise margin ( Supplementary Fig. S3C ), which is large compared with the low hysteresis, prerequisites for realizing larger and more complex integrated circuits. Figure 2: Flexible NCIC inverter constructed from NC-FETs. ( a ) Photograph and ( b ) circuit schematic of saturated load inverters. (1) Load NC-FET and (2) driver NC-FET. ( c ) Graphical analysis of constituent driver (black) and load (red) NC-FET output characteristics, sweeping in forward and reverse, comprising the NCIC inverter, and ( d ) the corresponding voltage transfer characteristics (black, left axis) and gain characteristics (blue, right axis) of the NCIC inverter sweeping forward and reverse at a supply voltage of 2 V ( V DD ). GND, ground. Full size image NC integrated amplifiers In Fig. 3a we demonstrate typical characteristics of the NCIC inverter operating as a common source with active load voltage amplifier. A 50-Hz, 100-mV sinusoidal signal is superimposed on a 0.6-V DC bias at the input (black). The output waveform (blue) is a replica of the input signal that is linearly amplified with no waveform distortion, is sinusoidally varying about a DC output voltage of 0.95 V as anticipated from the inverter’s VTC, and exhibits a 180° phase shift as expected from a common-source gain stage. The measured frequency response of the voltage amplifier has a 3-dB bandwidth (70.7% magnitude of the maximum gain of 4.59 dB) of 900 Hz ( Fig. 3b ), which is limited by parasitic capacitance in our current circuit design. We studied the single-time-constant network in the voltage amplifier and estimated a 3-dB bandwidth of 1.4 kHz ( Supplementary Fig. S4 and Discussion). 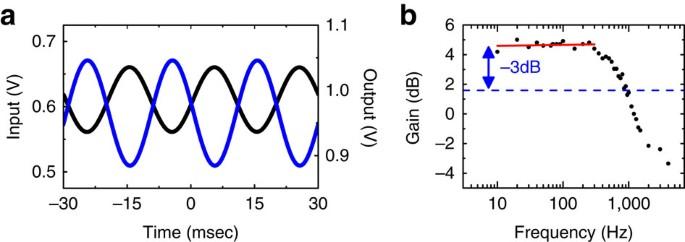Figure 3: Flexible NCIC amplifier and Bode plot. (a) Output waveform (blue, right axis) of NCIC voltage amplifier in response to a 50-Hz, 100-mV sinusoidal input on a 0.6-V DC bias (black, left axis). (b) Frequency response of a voltage amplifier (black circles). A linear fit (red solid line) shows a 4.59-dB voltage gain at low frequency, which is used to find the 3-dB bandwidth (blue dashed line). Figure 3: Flexible NCIC amplifier and Bode plot. ( a ) Output waveform (blue, right axis) of NCIC voltage amplifier in response to a 50-Hz, 100-mV sinusoidal input on a 0.6-V DC bias (black, left axis). ( b ) Frequency response of a voltage amplifier (black circles). A linear fit (red solid line) shows a 4.59-dB voltage gain at low frequency, which is used to find the 3-dB bandwidth (blue dashed line). Full size image NC integrated ring oscillators Building on the CdSe NCIC inverter as a logic switch, we integrated multiple inverter stages to construct the first NCIC ring oscillators. Using the same processes for circuit fabrication and VIA integration described for the inverter and amplifier, five-stage ring oscillators (ten NC-FETs) were fabricated over areas of 2 cm × 6 cm on flexible plastic ( Fig. 4a ). The circuit layout of the ring oscillator is depicted in Fig. 4b , showing the output of the fifth inverter stage connected to the input of the first inverter stage of the oscillator, and an additional sixth inverter used as a buffer stage to minimize the load and interconnect capacitances. 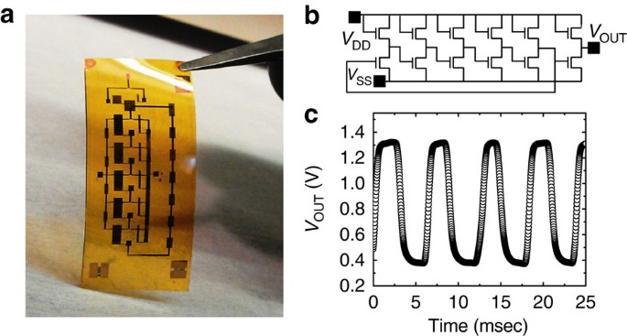Figure 4: Flexible NCIC ring oscillator constructed from NCIC inverters. (a) Photograph, (b) circuit schematic and (c) output characteristics of a five-stage NCIC ring oscillator with a sixth-stage buffer operating at a supply voltage of 2 V (VDD) with a frequency of 165 Hz. Figure 4c shows the output characteristics of a five-stage NCIC ring oscillator. The solution-deposited NC-FETs fabricated on plastic substrates form devices with uniform parameters over large areas to operate in concert as required to realize ring oscillators. The constituent NCIC inverter stages have adequate noise margin to support signal propagation through logic switching between ‘0’ (low) and ‘1’(high). At the low 2 V supply voltages, the ring oscillator output characteristic has no distortion across the 1 V rail-to-rail swing, spanning 67% of the output swing or 50% of the supply voltage. The oscillation frequency is ~165 Hz, that is, the signal delay per inverter is 606 μs. Similar to the amplifier, the measured frequency of the ring oscillator is limited by parasitic capacitances rather than by the intrinsic properties of the NC thin film. We estimated the signal delay per stage of the constituent inverters in the five-stage ring oscillator to be 170 μs ( Supplementary Figs. S5, S6 and Discussion) and is the first reported NC-FET-based ring oscillator. Figure 4: Flexible NCIC ring oscillator constructed from NCIC inverters. ( a ) Photograph, ( b ) circuit schematic and ( c ) output characteristics of a five-stage NCIC ring oscillator with a sixth-stage buffer operating at a supply voltage of 2 V ( V DD ) with a frequency of 165 Hz. Full size image The switching speed of the NCIC ring oscillator, which successfully operates at desired low-supply voltages, is comparable to other emerging solution-processable materials with similar channel lengths (40 μm) and low-voltage operation [31] , [32] , suggesting that colloidal semiconductor NC inks form a promising class for low-cost, thin-film analogue and digital electronics. The switching speeds is sufficient for sensor and display applications [33] , [34] , [35] . Faster switching times may be realized by designing circuits with shorter channel lengths and minimizing the parasitic capacitance. Improved fabrication techniques to achieve better alignment or to even develop self-aligned [36] , [37] , [38] structures will minimize parasitic capacitances to the femto Farad scale, promising not only faster switching but CdSe NCIC voltage amplifiers with MHz bandwidths. In conclusion we report the first NCICs, demonstrating low-voltage NCIC inverters, amplifiers and ring oscillators constructed from multiple high-performance NC-FET building blocks. By taking advantage of the non-corrosive thiocyanate ligand and doping of the CdSe NC thin film by mild thermal annealing, we fabricated high-performance NC-FETs and NCICs from colloidal NC inks over large areas on flexible plastics. The small variation in device parameters and large-scale uniformity of our solution-processed NC-FETs enabled functional NCIC circuits for both analogue and digital applications. Recent demonstrations of more sophisticated pseudo-complementary metal-oxide semiconductor circuits based on unipolar devices may be applied to improve the performance of these flexible NCICs [39] . With continued advances in NC ligand chemistry and doping, this class of solution-processable materials promises to grow beyond unipolar circuits to complementary metal-oxide semiconductor-based NCICs constructed from high-performance n - and p -type NC-FETs from the wide range of available colloidal NC ink chemistries. Materials Anhydrous solvents (highest grade available) were purchased from Acros, or purged and dried by standard methods. Ammonium thiocyanate (Acros, 99.8%+) was recrystallized from dry alcohol. Trioctylphosphine oxide (90%), tributylphosphine (97%), octadecylamine (99%) and selenium shot (99.99%) were purchased from Sigma-Aldrich. Cadmium stearate was purchased from MP Biomedicals. Kapton was purchased from DuPont. CdSe NC synthesis Cadmium selenide NCs were synthesized following a modified literature procedure [40] : 20 g trioctylphosphine oxide, 20 g octadecylamine and 2.10 g cadmium stearate were held under vacuum for 1 h at 120 °C, then heated to 320 °C under nitrogen, then 10.0 ml 1.25 M selenium in tributylphosphine solution was injected. Particle growth continued at 290 °C for 15 min. The peak of the first absorption maximum ranged from 580 to 583 nm across several independently synthesized batches. Ligand exchange with ammonium thiocyanate The exchange was performed in nitrogen atmosphere based on our previously published procedure [16] , [20] , and optimized for each individual batch of NCs. Typically, 1 ml of NH 4 SCN ranging in concentration from 100 to 250 mM in acetone was combined with 2 ml of CdSe NCs dispersed in hexane at an optical density of 5–10 cm −3 at the first excitionic absorption feature. The mixture was stirred with a vortexing mixer at 3,000 r.p.m. for 2 min, with complete flocculation observed within seconds. The slurry was centrifuged at 3,000 g for 1 min and the clear, colourless supernatant discarded. Tetrahydrofuran (2 ml) was added and the slurry mixed at 3,000 r.p.m. for 2 min, centrifuged at 3,000 g for 1 min and the clear, colourless supernatant discarded once more. Toluene (2 ml) was added and the slurry mixed at 3,000 r.p.m. for 1 min, centrifuged at 3,000 g for 1 min and the clear, colourless supernatant discarded. Dimethylformamide was added to the pellet to the desired concentration and the mixture was gently agitated until the NCs were fully dispersed. Flexible device fabrication N -type unipolar NC-FETs and NCICs (inverters, amplifiers and ring oscillators) were fabricated on either 25- or 50-μm thick preshrunk, Al 2 O 3 encapsulated polyimide substrates with thermally deposited 20-nm Al gate patterns. A Cambridge Nanotech Savannah 200 system was used to deposit Al 2 O 3 at 250 °C, using trimethylaluminum and water precursors. For integrated circuits, a subsequent VIA shadow mask was microscopically aligned and 60 nm of Au was thermally deposited to pattern the VIAs and integrate device layers. Both the FETs (only gate) and integrated circuits (both gate and VIA) were exposed to an oxygen plasma (75 mTorr, 100 W, 10 min) in a turbo-pumped parallel-plate reactive ion etcher at a base pressure of 3 × 10 −6 Torr to selectively increase the thickness of the native Al 2 O 3 atop the Al lines, but grew an unstable oxide atop Au VIAs in NCICs [28] , [29] . ALD Al 2 O 3 then selectively deposits a high-quality oxide atop the Al, but not atop the Au VIAs in NCICs, which still retain conductivity after ALD, as verified experimentally. Thiocyanate-exchanged CdSe NCs dispersed in dimethylformamide were then spincast uniformly atop the flexible substrates. A dispersion with an optical density of 40 was filtered through a 0.2-μm polytetrafluoroethylene filter and spincast at 500 r.p.m. for 30 s, followed by 800 r.p.m. for 30 s to yield dense, crack-free uniform NC thin films. In/Au electrodes were thermally evaporated through a shadow mask to either form FETs or integrated circuits in a nitrogen glovebox with an integrated evaporator. Devices were annealed in a nitrogen atmosphere for 10 min at 250 °C. FET and NCIC device measurements FET device characterization was performed on a Model 4156C semiconductor parameter analyser (Agilent) in combination with a Karl Suss PM5 probe station mounted in a nitrogen glovebox. Capacitance measurements (metal/dielectric/metal) were done using a Hewlett-Packard 4276 A LCZ metre. Inverter, amplifier and ring oscillator measurements were carried out using an oscilloscope from Tektronix, 33220 A waveform generator from Agilent, and a low-noise JEFT-input operational amplifier as the unity gain buffer. How to cite this article: Kim, D. K. et al . Flexible and low-voltage integrated circuits constructed from high-performance nanocrystal transistors. Nat. Commun . 3:1216 doi: 10.1038/ncomms2218 (2012).